Faradaic junction and isoenergetic charge transfer mechanism on semiconductor/semiconductor interfaces Energy band alignment theory has been widely used to understand interface charge transfer in semiconductor/semiconductor heterojunctions for solar conversion or storage, such as quantum-dot sensitized solar cells, perovskite solar cells and photo(electro)catalysis. However, abnormally high open-circuit voltage and charge separation efficiency in these applications cannot be explained by the classic theory. Here, we demonstrate a Faradaic junction theory with isoenergetic charge transfer at semiconductor/semiconductor interface. Such Faradaic junction involves coupled electron and ion transfer, which is substantively different from the classic band alignment theory only involving electron transfer. The Faradaic junction theory can be used to explain these abnormal results in previous studies. Moreover, the characteristic of zero energy loss of charge transfer in a Faradaic junction also can provide a possibility to design a solar conversion device with a large open-circuit voltage beyond the Shockley-Queisser limit by the band alignment theory. Since an energy band-alignment theory on p–n junctions was first proposed in 1949 [1] (Supplementary Fig. 1 ), a Si solar cell was developed to convert solar energy to electricity [2] . According to the band-alignment theory, Shockley and Queisser proposed a method to calculate the efficiency limit of a p–n solar cell, which has been a guideline in this field [3] . Thereafter, several emerging low-cost semiconductor/semiconductor junctions, such as quantum-dot-sensitized solar cells [4] , [5] , [6] and perovskite solar cells [7] , [8] , [9] , [10] , have been widely used for solar conversion. The band-alignment theory has also been used to calculate theoretical photovoltages of these emerging solar cells. For instance, a theoretical open-circuit voltage (V OC ) in a quantum-dot-sensitized solar cell (Supplementary Fig. 2a ) can be obtained from the difference between the conduction-band position of electron-transporting layer and redox potential [6] . Out of the expectation, some recent studies suggest that the experimental value of V OC is higher than the theoretical value in a quantum-dot-sensitized solar cell. Moreover, the V OC value changes with altering a quantum-dot sensitizer, but keeps constant with altering an electron-transporting material. These results are evidently inconsistent with the classic band-alignment theory [11] , [12] . Similar phenomena have also been observed in perovskite solar cells, in which the V OC value is only dependent on the band position of a perovskite absorber and a hole-transporting layer, not on an electron-transporting layer (Supplementary Fig. 2b ) [10] . Such abnormal V OC of a quantum-dot-sensitized or perovskite solar cell does not follow the classic band-alignment theory, which is still unclear to date. Moreover, semiconductor/semiconductor heterojunctions have been widely used to improve photocatalytic [13] , [14] , [15] , [16] , [17] or photoelectrocatalytic [18] , [19] , [20] performance. Two kinds of different interface charge-transfer mechanisms based on energy band alignment theory, type-II (Supplementary Fig. 2c ) and direct Z-scheme heterojunction (Supplementary Fig. 2d ), have been proposed to explain improved solar-conversion efficiency. In a type-II heterojunction, charge separation efficiency and photocurrent are enhanced significantly, which is mainly due to the built-in electric field at the interface. It is worthy to note that the charge separation in type-II heterojunction would decrease both reduction potential of electrons and oxidation potential of holes after interface charge transfer, and thereby leads to obvious photovoltage loss. However, some recent studies suggest that no energy loss of electrons is observed after interface charge transfer [17] , [21] . Therefore, a direct Z-scheme heterojunction mechanism was proposed to explain this phenomenon. For example, in a TiO 2 /CdS direct Z-scheme heterojunction, the electrons in the conduction band of TiO 2 would recombine with the holes in the valence band of CdS, while the holes in TiO 2 and the electrons in CdS can thus maintain their high oxidization and reduction potentials, respectively. However, no electrons could be photoexcited in TiO 2 under visible-light irradiation, which would result in less enhancement in the performance of a TiO 2 /CdS heterojunction. Nevertheless, remarkable enhancement on the photocatalytic performance of TiO 2 /CdS Z-scheme heterojunction was observed under both the full-arc and visible-light illumination [22] . The inconsistent results aforementioned suggest that the classic band-alignment theory is not suitable to describe this abnormal high V OC and charge-separation efficiency. Therefore, it is highly desirable to propose a theory to comprehend the interface charge transfer in these semiconductor/semiconductor junctions. Herein, by using a TiO 2 /CdS junction as a model, we investigated interface charge-transfer mechanism by in situ XPS, (quasi) in situ UV–vis, (quasi) in situ Raman, and electrochemical-impedance spectroscopy (EIS). Accordingly, we find that a TiO 2 /CdS heterojunction is a Faradaic junction, which is totally different from classic type-II or Z-scheme heterojunction. When photogenerated electrons in the conduction band of CdS inject into TiO 2 with H + ions from electrolyte, an intrinsic Faradaic layer on the surface of TiO 2 is reduced. The fast Faradaic reaction leads to much higher charge-separation efficiency in the TiO 2 /CdS Faradaic junction. The semiconductor/semiconductor Faradaic junction is also different from a semiconductor/farador junction in previous studies and few people consider a semiconductor as a farador with redox characteristic [23] , [24] . Very importantly, we also find the characteristic of isoenergetic interfacial charge transfer in the TiO 2 /CdS Faradaic junction, which can keep high reduction potential of the electrons in the semiconductor with higher conduction band. The Faradaic junction theory on semiconductor/semiconductor interface can be used to explain all these inconsistent results aforementioned in solar cells and photo(electro)catalysis fields. The theory is different from the classic band-alignment theory that was proposed over 70 years ago, which also provides a possibility to design a solar-conversion or storage device with a high V OC even beyond the Shockley–Queisser limit. Characterization and photoelectrochemical performance of TiO 2 /CdS A TiO 2 /CdS heterojunction was deposited on a FTO substrate by hydrothermal and successive ionic-layer adsorption and reaction method. Single TiO 2 and CdS electrode were also prepared as reference samples. Supplementary Fig. 3 and Fig. 1a indicate the scanning electron microscope (SEM) and transmission electron microscope (TEM) images of a TiO 2 /CdS heterojunction. CdS particles are uniformly coated on TiO 2 single-crystal nanorod arrays. The lattice spacing of 0.32 nm and 0.29 nm corresponds to the (110) and (001) of rutile TiO 2 , respectively. The observed 0.337-nm fringes on the surface of TiO 2 nanorod correspond to the (111) of CdS. 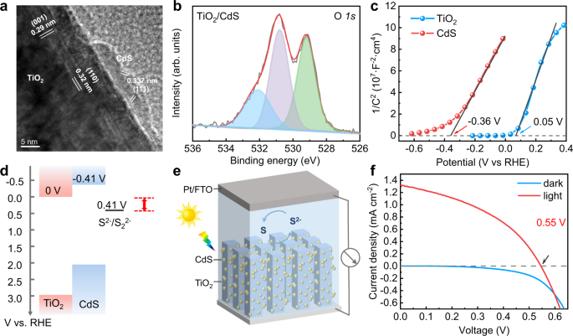Fig. 1: Characterization and VOCof TiO2/CdS. aA TEM image of TiO2/CdS, (b) XPS spectra of O 1 s of TiO2/CdS, (c) Mott–Schottky plots of TiO2and CdS in 1 M Na2S aqueous solution, (d) band positions of a TiO2/CdS heterojunction and redox potential of S2−/S, (e) a schematic diagram of a TiO2/CdS quantum-dot-sensitized solar cell, and (f) I–V curves of TiO2/CdS quantum-dot-sensitized solar cells under illumination and in the dark. Electrolyte: 0.5 M Na2S, 2 M S, and 0.2 M KCl in water/methanol (3:7 by volume). Light source: a Xe lamp with an AM 1.5 sunlight-simulator filter, light intensity: 100 mW/cm2. Figure 1b and Supplementary Fig. 4 indicate the X-ray photoelectron spectroscopy (XPS) patterns of TiO 2 /CdS. The binding energies of Ti 4+ , Cd 2+ , and S 2− peaks are observed on the surface of the sample, respectively. Similar to previous studies, the binding energies (529.2 eV, 530.9 eV, and 532.1 eV) of O 1 s are observed and assigned to the lattice O 2− , lattice OH − , and adsorbed H 2 O molecules, which suggests that there is indeed a TiO 2−x (OH) 2x layer on the surface of TiO 2 [25] . Fig. 1: Characterization and V OC of TiO 2 /CdS. a A TEM image of TiO 2 /CdS, ( b ) XPS spectra of O 1 s of TiO 2 /CdS, ( c ) Mott–Schottky plots of TiO 2 and CdS in 1 M Na 2 S aqueous solution, ( d ) band positions of a TiO 2 /CdS heterojunction and redox potential of S 2− /S, ( e ) a schematic diagram of a TiO 2 /CdS quantum-dot-sensitized solar cell, and ( f ) I–V curves of TiO 2 /CdS quantum-dot-sensitized solar cells under illumination and in the dark. Electrolyte: 0.5 M Na 2 S, 2 M S, and 0.2 M KCl in water/methanol (3:7 by volume). Light source: a Xe lamp with an AM 1.5 sunlight-simulator filter, light intensity: 100 mW/cm 2 . Full size image In order to investigate the relationship between the V OC of a solar cell and band alignment of different materials, the flat band potentials of TiO 2 and CdS were measured by Mott–Schottky (M–S) method and the results are 0.05 V RHE and −0.36 V RHE (Fig. 1c ). Generally, the conduction-band position is about 0.05 V higher than the flat-band potential [26] . Therefore, the conduction-band positions of TiO 2 and CdS are 0 V RHE and −0.41 V RHE , respectively, which are in good agreement with previous reports [27] , [28] . Similar band positions of TiO 2 and CdS are also obtained by ultraviolet photoelectron spectroscopy and UV–visible absorption spectroscopy methods (Supplementary Fig. 5 and Table 1 ). Moreover, the redox potential of S 2− /S was also measured as 0.41 V RHE on a Pt/FTO electrode by cyclic voltammetry (CV) method (Supplementary Fig. 6 ). According to the results, the band positions of CdS, TiO 2 , and redox potential of S 2− /S are plotted in Fig. 1d . From a classic band-alignment theory, a maximum theoretical V OC of a CdS quantum-dot-sensitized solar cell is 0.41 V. In order to investigate the experimental V OC , a solar cell was assembled with a TiO 2 /CdS heterojunction as a photoanode, a Pt/FTO as a counter electrode, and polysulfide solution as electrolyte (Fig. 1e ). The I–V curves of the solar cell were measured under illumination and in the dark, as shown in Fig. 1f . A V OC of 0.55 V is obtained from the I–V curve, which is further confirmed by open-circuit potential method (Supplementary Fig. 7 ). The experimental V OC is close to previously reported values [29] and is higher than the theoretical value of 0.41 V. The V OC of a quantum-dot-sensitized solar cell cannot be explained by classic band-alignment theory. Experimental evidence on a Faradaic reaction at TiO 2 /CdS interface In order to clarify the reasons for abnormally high V OC , we investigated interface charge-transfer mechanism in TiO 2 /CdS by in situ XPS, (quasi) in situ UV–vis, (quasi) in situ Raman, and EIS method. 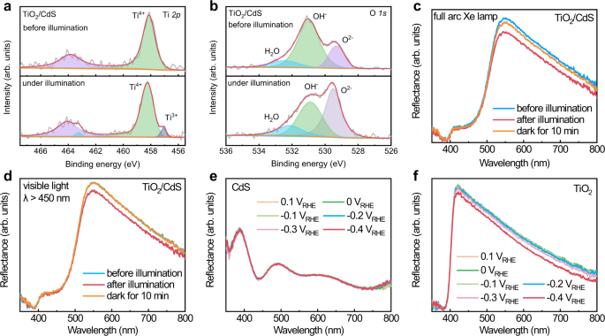Fig. 2: Charge-transfer process at TiO2/CdS interface. In situ XPS spectra of Ti 2p (a) and O 1 s (b) in TiO2/CdS in the dark and under full arc Xe lamp illumination, quasi in situ UV–vis reflectance spectra of TiO2/CdS in 1 M Na2S aqueous solution before and after illumination under full-arc Xe lamp (c) and visible light ofλ> 450 nm (d), and in situ UV–vis reflectance spectra of CdS (e) and TiO2(f) in 1 M Na2S aqueous solution at different potentials in the dark. In the dark, only Ti 4+ is observed on the surface of TiO 2 /CdS, while some Ti 4+ is reduced into Ti 3+ under illumination (Fig. 2a ). The decrease of the ratio of lattice OH − /lattice O 2− under illumination comes from oxidation of OH − by photogenerated holes in TiO 2 (Fig. 2b ). Moreover, the binding energies of Cd 3d and S 2p do not change under illumination (Supplementary Fig. 8 ), which suggests that a chemical reaction only happens on the surface of TiO 2 rather than CdS. In order to further investigate the reaction on the surface of TiO 2 /CdS, quasi in situ UV–vis reflectance spectra of a TiO 2 /CdS heterojunction were measured under open-circuit condition before and after full-arc Xe lamp illumination and the results are shown in Fig. 2c . After illumination, TiO 2 /CdS indicate lower reflectance at the wavelength range of 520–800 nm . In contrast, reflectance spectra of a single CdS and TiO 2 electrode do not change after illumination (Supplementary Fig. 9 ). Moreover, a PL peak of CdS at 690 nm [30] is quenched by contacting with TiO 2 (Supplementary Fig. 10 ), which suggests that interface charge transfer happens between CdS and TiO 2 . The lower reflectance after illumination possibly comes from charge-transfer-induced change of TiO 2 /CdS. The same change trend of reflectance spectra was also observed when the TiO 2 /CdS was illuminated under visible light ( λ > 450 nm), though TiO 2 was not excited (Fig. 2d ). Therefore, the visible light can still lead to the change of TiO 2 /CdS. In order to identify the change of reflectance from TiO 2 or CdS, we measured in situ reflectance spectra of a single CdS and TiO 2 electrode at different potentials in the dark (Fig. 2e, f ). The reflectance spectra of a CdS electrode do not change at the potential range from −0.4 V RHE to 0.1 V RHE , while the reflectance spectra of a TiO 2 electrode decrease at the potentials negative than −0.2 V RHE , which comes from a reduction reaction of an intrinsic Faradaic layer of TiO 2−x (OH) 2x (Ti +4 O 2−x (OH) 2x +H + + e − ↔ Ti +3 O 1−x (OH) 2x+1 ) on the surface of TiO 2 [31] . The electron concentration in the surface Faradaic layer of TiO 2 increases remarkably after reduction and leads to plasma-resonance absorption of free electrons at long wavelength [32] . Therefore, the lower reflectance in TiO 2 /CdS after illumination suggests that a reduction Faradaic reaction happens on the surface of TiO 2 . Fig. 2: Charge-transfer process at TiO 2 /CdS interface. In situ XPS spectra of Ti 2p ( a ) and O 1 s ( b ) in TiO 2 /CdS in the dark and under full arc Xe lamp illumination, quasi in situ UV–vis reflectance spectra of TiO 2 /CdS in 1 M Na 2 S aqueous solution before and after illumination under full-arc Xe lamp ( c ) and visible light of λ > 450 nm ( d ), and in situ UV–vis reflectance spectra of CdS ( e ) and TiO 2 ( f ) in 1 M Na 2 S aqueous solution at different potentials in the dark. Full size image In order to make clear why the Faradaic reaction happens only on the surface of TiO 2 , not CdS, CV and galvanostatic charge–discharge (GCD) curves of TiO 2 and CdS were measured and the results are shown in Supplementary Fig. 11 . Obvious hysteresis loop of a Faradaic reaction is observed in the CV curve of TiO 2 but not in CdS (Supplementary Fig. 11a ). The Faradaic potential window of TiO 2−x (OH) 2x is further determined at the potential range from −0.4 V RHE to 0.1 V RHE by GCD method, while negligible Faradaic charge and discharge process is observed on CdS (Supplementary Fig. 11b ). The results are in good agreement with previous study [31] . Therefore, a Faradaic reaction happens more easily on TiO 2 than on CdS at the same reduction potential. Quasi in situ Raman spectroscopy was also used to investigate interface changes [33] in a TiO 2 /CdS heterojunction under illumination and the results are shown in Fig. 3a . The Raman peak intensity of TiO 2 /CdS decreases after illumination, which comes from the formation of amorphous Ti +3 O 1−x (OH) 2x+1 on the surface of TiO 2 [34] . In contrast, the Raman peak intensities of single CdS and TiO 2 do not change after illumination, which further confirm the interface charge transfer in TiO 2 /CdS (Supplementary Fig. 12 ). Similar to in situ UV–vis characterization in Fig. 2b and c, in situ Raman spectra of CdS and TiO 2 were also measured at different potentials in the dark. The Raman peak intensity of CdS changes slightly (Fig. 3b ), but the Raman peak intensity of TiO 2 decreases with decreasing potentials (Fig. 3c ). Therefore, the Raman spectra also suggest that charge transfer induced surface changes not on CdS but on TiO 2 under illumination. Moreover, no obvious XRD change is observed in TiO 2 /CdS before and after illumination (Supplementary Fig. 13 ), which further confirms that the Faradaic reaction only happens on the surface of TiO 2 , not the bulk. In order to investigate the reaction process of H ions in the intrinsic Faradaic layer, isotope-labeling experiments by using D 2 O as a solvent were carried out and time-of-flight secondary-ion mass spectrometry (TOF-SIMS) was used to analyze depth profiles of D ions in the Faradaic junction before and after illumination. The results are shown in Fig. 3d . Ti ions are observed at the depth with sputtering time of 0–100 s and the distribution does not change before and after illumination. For D-ion depth profile, only possible adsorption of D ions on the surface of the sample before illumination, no D ions can be observed at the depth with sputtering time >10 s. After illumination, remarkably enhanced intensity of D ions is observed, and the distribution is in good agreement with the Ti ions, which suggest that D ions in the electrolyte insert into TiO 2 under illumination. The concentration of H ions has significant effects on the efficiency of the TiO 2 /CdS heterojunction (Supplementary Fig. 14 ), which further supports the Faradaic junction mechanism at TiO 2 /CdS interface. Moreover, we find that the Faradaic reaction at TiO 2 /CdS interface not only happens in liquid phase, but also in gas-phase and solid-phase surroundings (Supplementary Figs. 15 and 16 ). Therefore, the Faradaic junction mechanism is universal to understand interface charge transfer in liquid photoelectrochemistry, gas photocatalysis, or solid-state solar cells. Fig. 3: Interface change and ion-depth profiles in TiO 2 /CdS under illumination. a Quasi in situ Raman spectra of TiO 2 /CdS before and after illumination under full-arc Xe lamp, in situ Raman spectra of CdS ( b ) and TiO 2 ( c ) in 1 M Na 2 S aqueous solution at different potentials in the dark, ( d ) secondary ion intensities of Ti and D ions in a TiO 2 /CdS junction in the electrolyte (1 M Na 2 S in D 2 O solution) before and after illumination for 10 min, electrochemical-impedance spectroscopy @0.4 V RHE of TiO 2 /CdS in 1 M Na 2 S aqueous solution with air ( e ) and with Ar ( f ) before and after illumination under full-arc Xe lamp. Full size image Electrochemical-impedance spectroscopy (EIS) method was also used to investigate interface charge transfer in TiO 2 /CdS and the results are shown in Fig. 3e . In the dark, a TiO 2 /CdS heterojunction indicates similar EIS spectra with single TiO 2 , not CdS (Supplementary Fig. 17 ). Since CdS particles do not cover TiO 2 nanorods completely and TiO 2 contacts with electrolyte directly, the impedance spectra of TiO 2 /CdS mainly reflect the property of TiO 2 . The semicircle at low frequency of TiO 2 /CdS decreases obviously after illumination, which comes from the lower charge-transfer resistance in the TiO 2 /electrolyte interface [35] . In contrast, the impedance circle of single TiO 2 and CdS does not change after the same illumination (Supplementary Fig. 18 ). Therefore, the decreased impedance semicircle of TiO 2 /CdS after illumination comes from the reduction reaction of an intrinsic Faradaic layer of TiO 2−x (OH) 2x by photogenerated electrons from CdS . Moreover, since a Faradaic reaction is reversible, we also observed recovery process of UV–vis (Fig. 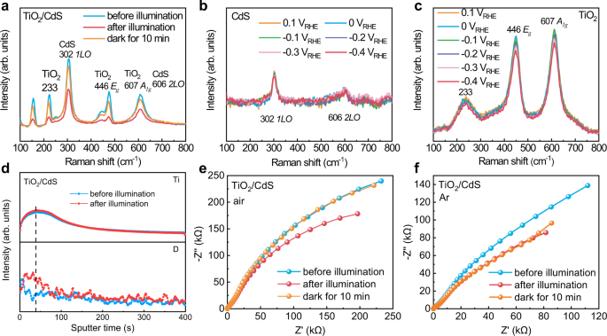Fig. 3: Interface change and ion-depth profiles in TiO2/CdS under illumination. aQuasi in situ Raman spectra of TiO2/CdS before and after illumination under full-arc Xe lamp, in situ Raman spectra of CdS (b) and TiO2(c) in 1 M Na2S aqueous solution at different potentials in the dark, (d) secondary ion intensities of Ti and D ions in a TiO2/CdS junction in the electrolyte (1 M Na2S in D2O solution) before and after illumination for 10 min, electrochemical-impedance spectroscopy @0.4 VRHEof TiO2/CdS in 1 M Na2S aqueous solution with air (e) and with Ar (f) before and after illumination under full-arc Xe lamp. 2c–d ), Raman spectra (Fig. 3a ) and EIS spectra (Fig. 3e ) of TiO 2 /CdS when light was off and the sample was kept in electrolyte with air for 10 min. In contrast, no recovery process of EIS spectra was observed in the same electrolyte with Ar bubbling (Fig. 3f ). The results suggest that the reduced intrinsic Faradaic layer on the surface of TiO 2 can be reoxidized by dissolved oxygen in the electrolyte. A proposed mechanism Subsequently, we further study interface charge transfer characteristics of a TiO 2 /CdS Faradaic junction by linear-sweep voltammetry (LSV) and open-circuit potential (OCP) electrochemical methods. 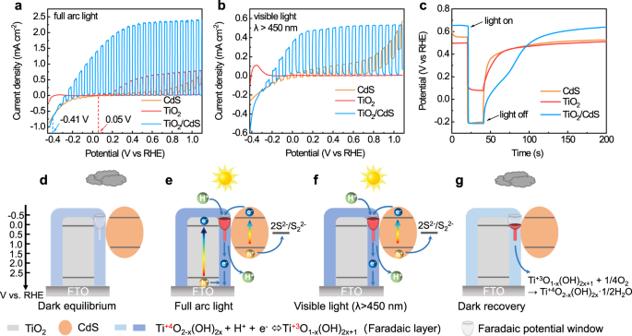Fig. 4: Characteristic and mechanism of isoenergetic charge transfer in a Faradaic junction. Linear-sweep voltammetry curves of TiO2, CdS and TiO2/CdS in 1 M Na2S aqueous solution under chopped full-arc Xe lamp illumination without (a) and with (b) a filter (wavelength >450 nm); (c) open-circuit potential of TiO2, CdS, and TiO2/CdS in 1 M Na2S aqueous solution with air in the dark and under illumination; (d–g) interface charge-transfer mechanisms in a TiO2/CdS heterojunction in the dark and under illumination. Figure 4a and b shows LSV curves of TiO 2 , CdS and TiO 2 /CdS in 1 M Na 2 S aqueous solution under full-arc and visible-light illumination, respectively. The photocurrent-onset potentials of TiO 2 , CdS, and TiO 2 /CdS are 0 V RHE , −0.41 V RHE (Supplementary Fig. 19 ), and −0.41 V RHE , respectively, which are in good agreement with the conduction-band position in Fig. 1d . The onset potential of TiO 2 /CdS is the same to that of CdS, not TiO 2 , which suggests that the photogenerated electrons in CdS can be transferred to TiO 2 without energy loss. Moreover, the TiO 2 /CdS indicates much higher stable photocurrent than those of TiO 2 and CdS at different potentials, especially close to the onset potential of CdS (Supplementary Fig. 20 ). The results suggest that the TiO 2 /CdS heterojunction can not only keep the high reduction energy of photogenerated electrons of CdS, but also improve separation efficiency of photogenerated carriers simultaneously. An OCP method was also used to investigate interface charge-transfer process in the TiO 2 /CdS heterojunction (Fig. 4c ). TiO 2 , CdS, and TiO 2 /CdS indicate different open-circuit potentials in the dark, which comes from chemical equilibrium between a sample surface and redox couples in the electrolyte. Under illumination, open-circuit potentials of the three samples are 0.07 V RHE , −0.2 V RHE , and −0.2 V RHE , respectively. The open-circuit potential of TiO 2 under illumination is close to its onset potential. However, the open-circuit potential of CdS under illumination is 210 mV positive than its onset potential. The OCP is a potential with zero current, which indicates equilibrium potential of photooxidation for S 2− and dark reduction of S on a sample. There is much higher dark-reduction current of S than photooxidation for S 2− on CdS at the potential negative than −0.2 V RHE (Supplementary Fig. 21a ), which leads to the OCP of CdS pinning at −0.2 V RHE . In contrast, no obvious dark-reduction current of S is observed on TiO 2 (Supplementary Fig. 21b ). Therefore, the OCP of CdS under illumination is different from its onset potential, while the OCP of TiO 2 under illumination is close to the onset potential. The TiO 2 /CdS indicates the same open-circuit potential under illumination to that of CdS, which further confirms that transferred electrons from CdS to TiO 2 indicate the same energy to those in CdS. Moreover, when the light is off, slower decay process of OCP on TiO 2 comes from reoxidization of the reduced-surface Faradaic layer by oxygen in the electrolyte (Supplementary Fig. 22 ). A TiO 2 /CdS heterojunction indicates the slowest decay process of the open-circuit potential among the three samples when the light is off. It is because of much negative potential of the photogenerated electrons in TiO 2 /CdS than that of TiO 2 , which leads to deeper reduction of the intrinsic Faradaic layer. Therefore, a TiO 2 /CdS heterojunction indicates an unusual isoenergetic interface charge transfer by a Faradaic reaction under illumination. Fig. 4: Characteristic and mechanism of isoenergetic charge transfer in a Faradaic junction. Linear-sweep voltammetry curves of TiO 2 , CdS and TiO 2 /CdS in 1 M Na 2 S aqueous solution under chopped full-arc Xe lamp illumination without ( a ) and with ( b ) a filter (wavelength >450 nm); ( c ) open-circuit potential of TiO 2 , CdS, and TiO 2 /CdS in 1 M Na 2 S aqueous solution with air in the dark and under illumination; ( d – g ) interface charge-transfer mechanisms in a TiO 2 /CdS heterojunction in the dark and under illumination. Full size image According to the above results and analysis, we propose an interface charge-transfer mechanism in a TiO 2 /CdS heterojunction in Fig. 4 d–g. In the dark, there is an intrinsic Faradaic layer of Ti +4 O 2−x (OH) 2x at the interface of a TiO 2 /CdS heterojunction. The composition of the intrinsic Faradaic layer sensitively depends on potential and chemical equilibrium between a sample surface and redox couples in the electrolyte. Under illumination, photogenerated electrons in the conduction band of CdS transfer to TiO 2 , as well as H + from the electrolyte, which reduce the intrinsic Faradaic layer (Ti +4 O 2−x (OH) 2x ) and raise its fermi level to the same position with the conduction-band bottom of CdS. Therefore, isoenergetic interfacial charge transfer is observed in a TiO 2 /CdS junction under illumination. The resistance of the reduced Faradaic layer (Ti +3 O 1−x (OH) 2x+1 ) decreases remarkably and forms a short-circuit pathway for the electron transfer from the surface of TiO 2 to a FTO substrate directly, not through the bulk of TiO 2 (Fig. 4e ), which is different from type-II heterojunction (Supplementary Fig. 23 ). Under full arc illumination, both of TiO 2 and CdS are excited, the photogenerated electrons on TiO 2 transfer to the FTO substrate through the bulk of TiO 2 , and the photogenerated holes diffuse to the surface of TiO 2 and react with the reduced-surface Faradaic layer of Ti +3 O 1−x (OH) 2x+1 . Though a Faradaic reaction is observed at TiO 2 /CdS interface, the interface charge-transfer mechanism is also different from that in an indirect Z-scheme heterojunction with Au or redox shuttle as electron mediator (Supplementary Fig. 24 ) [36] . In a Faradaic junction, photogenerated electrons transfer from CdS to TiO 2 , however, reverse charge transfer direction in a Z-scheme junction. Under visible-light illumination (>450 nm), only CdS is excited (Fig. 4f ), the reduced Faradaic layer of Ti +3 O 1−x (OH) 2x+1 plays a role as a charge separator by a fast Faradaic reaction and an electron-transfer pathway, which can improve the photoelectrochemical performance of CdS. When the light is off, the reduced Faradaic layer can be oxidized by oxygen in the electrolyte and a reversible Faradaic reaction happens, which leads to the Fermi level recovering to the initial value before illumination (Fig. 4g ). Therefore, the interface charge-transfer mechanism in a TiO 2 /CdS heterojunction is neither type-II heterojunction nor Z-scheme heterojunction, but a Faradaic junction, in which the characteristic of zero-energy loss and high charge-separation efficiency can be obtained at the same time by a fast and reversible Faradaic reaction. In order to further investigate universality of the semiconductor/semiconductor Faradaic junction theory, we also prepared different oxide semiconductors (ZnO, Nb 2 O 5 , and Fe 2 O 3 ) to replace TiO 2 and constructed heterojunctions with CdS (Supplementary Figs. 26 and 27 ). Similar to TiO 2 /CdS, impedance semicircles of the ZnO/CdS, Nb 2 O 5 /CdS, and Fe 2 O 3 /CdS decrease after illumination, which also possibly come from reduction of intrinsic Faradaic layers of ZnO, Nb 2 O 5 and Fe 2 O 3 by photogenerated electrons from CdS (Supplementary Fig. 28 ). Moreover, ZnO/CdS and Nb 2 O 5 /CdS heterojunctions indicate close onset potentials to that of CdS. However, the onset potential of Fe 2 O 3 /CdS heterojunction indicates 0.56 V positive than that of CdS (Supplementary Figs. 29 – 30 ). These results suggest that isoenergetic charge transfer also happens at ZnO/CdS and Nb 2 O 5 /CdS interfaces, but not at Fe 2 O 3 /CdS interface. In order to explain this phenomenon, we measured the Faradaic potential windows of ZnO, Nb 2 O 5 , and Fe 2 O 3 and the results are plotted in Supplementary Fig. 31 . ZnO and Nb 2 O 5 indicate similar Faradaic potential windows to that of TiO 2 , while the Faradaic potential window of Fe 2 O 3 is 0.50 V positive than that of TiO 2 . When a potential negative than 0.03 V RHE is applied on a Fe 2 O 3 electrode, a corrosion reaction (Fe +3 O x (OH) 3−2x + 3H + + e − → Fe 2+ + (3−x)H 2 O) happens and Fe 2 O 3 is dissolved into the electrolyte (Supplementary Fig. 32 ). Therefore, when the photogenerated electrons in the conduction band of CdS transfer to ZnO and Nb 2 O 5 , the intrinsic Faradaic layers can be charged and their fermi levels can be raised to the same position with the conduction-band bottom of CdS. The results can explain the V OC dependent on a quantum-dot sensitizer but not on an electron-transporting material in quantum-dot-sensitized or perovskite solar cells [10] , [11] , [12] . However, when the photogenerated electrons in the conduction band of CdS transfer to Fe 2 O 3 , the photogenerated electrons will lead to dissolution of Fe 2 O 3 . Therefore, a prerequisite of isoenergetic charge transfer at semiconductor/semiconductor Faradaic interfaces is that the conduction-band position of an electron-donor semiconductor should overlap with a Faradaic potential window of an electron-acceptor semiconductor (Supplementary Fig. 33 ). In summary, we propose a Faradaic junction mechanism on a TiO 2 /CdS heterojunction, which is substantively different from classic band-alignment theory on a semiconductor/semiconductor junction. The Faradaic junction mechanism is observed not only in liquid-phase, but also in gas-phase and solid-phase surroundings. Moreover, we find that a TiO 2 /CdS Faradaic junction indicates unusual isoenergetic interface charge transfer, which can be used to explain abnormal photovoltages or reduction/oxidation potential in quantum dot/perovskite solar cells and photo(electro)catalysis. We also propose a prerequisite of isoenergetic charge transfer in semiconductor/semiconductor Faradaic junctions. The Faradaic junction theory can offer a different perspective to design semiconductors with suitable Faradaic potential windows, but not conventional band positions, for high-performance solar energy conversion and storage. Preparation of TiO 2 nanorod films TiO 2 nanorod films were prepared on FTO substrates by hydrothermal method [25] . Briefly, 15 mL of deionized water and 15 mL of HCl were mixed and stirred for 10 min. Then, 0.45 mL of titanium butoxide was added. The solution was transferred to a Teflon-lined steel autoclave with inserting FTO substrates in it. The hydrothermal reaction was conducted at 150 o C for 9 h. Finally, the deposited films were washed by deionized water and calcined at 450 o C for 1 h in air. Preparation of CdS on TiO 2 nanorod array by SILAR method CdS QDs were grown on the TiO 2 nanorod array by successive ionic-layer adsorption and reaction (SILAR) method [37] , [38] . Typically, the TiO 2 nanorod array films were immersed in Cd(CH 3 COO) 2 solution (0.1 M) for 2 min and rinsed with deionized water, and then immersed in Na 2 S solution (0.1 M) for another 2 min followed by another rinsing with deionized water. Such a SILAR cycle was repeated for 15 times to obtain TiO 2 /CdS samples. CdS on FTO substrates was also prepared by the same method as reference samples. Characterization of samples X-ray diffraction (XRD smartlab 9 kW) was used to characterize the crystal structures of the samples. Scanning electron microscope (SEM Nano Nova S230) and transmission electron microscope (TEM Tecnai G2 F20) were used to investigate the morphologies of the samples. X-ray photoelectron spectroscopy (XPS) was performed on a K-Alpha instrument operating with an Al Kα X-ray source. The binding energy was calibrated by C1s peak at 284.6 eV. Photoluminescence spectra (PL) of the samples were collected by a Renishaw InVia Raman Micro-PL system with a 375-nm He–Cd laser. Time-of-flight secondary-ion mass spectrometry (TOF-SIMS 5 iontof, PHI NanoTOFII) was used to analyze depth profiles of ions in the Faradaic junction before and after illumination. In situ characterization of samples In situ UV–vis reflection spectra (UV, Shimadzu UV-2550) and in situ Raman (Horiba T64000, excitation wavelength ~488 nm) in the dark were measured in a cell with a Pt wire and a saturated Ag/AgCl electrode as the counter and reference electrode, respectively. The electrolyte was 1 M Na 2 S aqueous solution (pH~13.3). An electrochemical analyzer (CHI 760e, Shanghai Chenhua) was used to control the potentials of the samples. Quasi in situ UV–vis reflection and Raman spectra were measured immediately after the photoelectrodes were illuminated by a Xe lamp in 1 M Na 2 S aqueous solution (pH~13.3) at an open-circuit potential. In situ X-ray photoelectron spectroscopy (Thermofisher Escalab 250Xi) was performed under a full-arc Xe lamp. The prepared TiO 2 /CdS sample was kept in the dark before the test. The sample was immersed in 0.5 M Na 2 SO 3 aqueous solution and dried in air. Before measurement, the sample was exposed to water vapor for 10 min, and then in situ XPS was measured on the sample in the dark and after 3-mins’ illumination. Photoelectrochemical measurement The photoelectrochemical properties of the films were investigated in a three-electrode cell using an electrochemical analyzer (CHI 760e, Shanghai Chenhua) under a Xe lamp with an AM 1.5 sunlight-simulator filter illumination (light intensity: 100 mW/cm2). A Pt mesh and a saturated Ag/AgCl electrode were used as a counter electrode and a reference electrode, respectively. The electrolyte was 1 M Na 2 S aqueous solution (pH~13.3). A reversible hydrogen electrode (RHE) potential was obtained by the following formula: V RHE = V Ag/AgCl + 0.059*pH + 0.197. The quantum-dot-sensitized solar cell full device was assembled by using TiO 2 /CdS as a photoelectrode and a Pt-sputtered FTO as a counter electrode. The electrolyte was 0.5 M Na 2 S, 2 M S, and 0.2 M KCl in water/methanol (3:7 by volume) [39] . The I–V curves of solid-state solar cells were measured by Keithley 2450. Reporting summary Further information on research design is available in the Nature Research Reporting Summary linked to this article.